The ZNF304-integrin axis protects against anoikis in cancer Ovarian cancer (OC) is a highly metastatic disease, but no effective strategies to target this process are currently available. Here, an integrative computational analysis of the Cancer Genome Atlas OC data set and experimental validation identifies a zinc finger transcription factor ZNF304 associated with OC metastasis. High tumoral ZNF304 expression is associated with poor overall survival in OC patients. Through reverse phase protein array analysis, we demonstrate that ZNF304 promotes multiple proto-oncogenic pathways important for cell survival, migration and invasion. ZNF304 transcriptionally regulates β1 integrin, which subsequently regulates Src/focal adhesion kinase and paxillin and prevents anoikis. In vivo delivery of ZNF304 siRNA by a dual assembly nanoparticle leads to sustained gene silencing for 14 days, increased anoikis and reduced tumour growth in orthotopic mouse models of OC. Taken together, ZNF304 is a transcriptional regulator of β1 integrin, promotes cancer cell survival and protects against anoikis in OC. Ovarian carcinoma (OC) has the highest mortality rate among gynecologic malignancies. In the United States in 2014, over 21,000 patients will be diagnosed with OC, and more than 14,000 will die [1] . The most common histological subtype is high-grade serous OC (HGSOC), which is associated with poor survival most likely due to the advanced stage of disease and widespread metastases at presentation, related to lack of early symptoms and detection. The rapid spread of HGSOC is based on its propensity to seed the peritoneal cavity, leading to ascites formation [2] , [3] ; this highlights the need for a deeper understanding of the molecular mechanisms that regulate OC growth and progression. The Cancer Genome Atlas (TCGA) is paving the way for new target identification that may influence pathophysiology and patient outcome. This data set provides a comprehensive genomic, epigenomic and a number of other analysis, which will assist in the detection of biological and clinically relevant information on HGSOC samples [4] . To identify new therapeutic targets and strategies, we carried out an integrative analysis of TCGA HGSOC data set [4] and gene profiles of ovarian and breast tumours to identify genes that are important for cancer metastasis. Among the genes identified, zinc finger protein 304 (ZNF304) was found to be the most highly associated with overall survival in HGSOC patients. ZNF304 is a transcription factor that belongs to the C2H2 zinc finger family. The member genes of this family represent the largest class of transcription factors in humans and, indeed, one of the largest gene families in mammals [5] . ZNF304 can be upregulated by activated Kirsten rat sarcoma viral oncogene homologue (KRAS) in KRAS-positive colorectal cancer cells and binds at the promoters of INK4-ARF and other CpG island methylator phenotype genes in colorectal cancer cells and in human embryonic stem cells [6] . However, the role of ZNF304 in metastasis and its downstream effectors are not well understood. This study demonstrates that ZNF304 regulates inside-out anoikis through the regulation of β1 integrin in OC cells, resulting in increased migration, proliferation and decreased anoikis. Using dual assembly nanoparticles (DANP) loaded with ZNF304 short interfering RNA (siRNA), we achieved long-term silencing after a single administration in orthotopic models of OC, which led to reduced tumour weight and number of nodules, recapitulating the in vitro findings. Thus, ZNF304 is an attractive target for OC therapy. ZNF304 in human HGSOC We first carried out an integrative computational analysis to identify genes that are important for cancer metastasis and that are upregulated in OC. As N-cadherin has been reported to play a critical role in invasion and anoikis resistance of cancer cells [7] , [8] , we first identified gene signatures in tumours with high N-cadherin expression in TCGA HGSOC data set. Of 16,869 genes that were upregulated in OC, 493 genes had a positive correlation with tumoral N-cadherin expression ( Fig. 1a ). Of these 493 genes, ciliary neurotrophic factor receptor ( CNTFR ); melanoma antigen family D, 1 ( MAGED1 ); nuclear receptor subfamily 2, group F, member 2 ( NR2F2 ) and ZNF304 were upregulated in invasive ovarian and breast tumour epithelium compared with normal ovarian [9] and breast epithelium [10] , respectively. 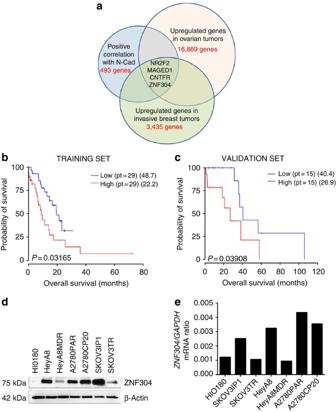Figure 1: Significance of zinc finger protein 304 expression in human ovarian carcinoma (OC). (a) Graphical representation of computational analysis using The Cancer Genome Atlas (TCGA) high-grade serous OC data set. (b) The probability of survival in OC patients analysed in the training set (two-third of cases;P<0.05, Log-rank test) and (c) in the validation set (one-third of cases;P<0.05, Log-rank test). Kaplan–Meier curves indicate that high ZNF304 expression is a predictor of poor overall survival in patients with OC (n=88,P=0.03, Log-rank test). (d) Western blot analysis of ZNF304 protein expression and (e) RT-PCR analysis of ZNF304 mRNA in six ovarian cancer cell lines and one non-transformed ovarian cell line (HIO180). Figure 1: Significance of zinc finger protein 304 expression in human ovarian carcinoma (OC). ( a ) Graphical representation of computational analysis using The Cancer Genome Atlas (TCGA) high-grade serous OC data set. ( b ) The probability of survival in OC patients analysed in the training set (two-third of cases; P <0.05, Log-rank test) and ( c ) in the validation set (one-third of cases; P <0.05, Log-rank test). Kaplan–Meier curves indicate that high ZNF304 expression is a predictor of poor overall survival in patients with OC ( n =88, P =0.03, Log-rank test). ( d ) Western blot analysis of ZNF304 protein expression and ( e ) RT-PCR analysis of ZNF304 mRNA in six ovarian cancer cell lines and one non-transformed ovarian cell line (HIO180). Full size image We then assessed the effect of tumoral expression on patient survival for these four genes using TCGA HGSOC data set ( Supplementary Fig. 1 ). For each gene, we randomly split the entire OC patient population into training (two-third of cases) and validation cohorts (one-third of cases). In both cohorts, patients were divided into sextiles according to mRNA expression, and the first and last sextiles were contrasted. Importantly, the relationships between overall survival and known prognostic factors such as age or residual disease were examined in both the training and the validation cohorts using a Cox proportional hazards model. Only ZNF304 was a significant factor in this analysis ( Fig. 1b,c ). In contrast, CNTFR (Training and validation sets; Supplementary Fig. 1a,b , respectively), MAGED1 (Training and validation sets; Supplementary Fig. 1c,d , respectively) and NR2F2 (Training and validation sets; Supplementary Fig. 1e,f , respectively) expression levels were not correlated with patient survival. Patients with high tumoral ZNF304 expression had significantly lower median overall survival than patients with low tumoral ZNF304 expression, Fig. 1b (training set, 22.2 versus 48.7 months, P =0.031, Log-rank test) and Fig. 1c (validation set, 40.4 versus 26.9 months, P =0.039, Log rank test). Based on these results, ZNF304 was selected for additional studies. Next, we examined protein expression levels of ZNF304 (75 kDa) by western blot analysis in six OC tumour cell lines and in HIO180 non-transformed ovarian epithelial cells ( Fig. 1d ). ZNF304 protein was highly expressed in all OC cells tested, but a lower expression was observed in the HIO180 cells. ZNF304 mRNA basal levels were high in four of the six OC cell lines ( Fig. 1e ). In addition, we analysed ZNF304 mRNA levels in patient normal distal fallopian tubes versus HIO180 and SKOV3IP1 cancer cells ( Supplementary Fig. 2 ). ZNF304 mRNA levels were similar between fallopian tube and HIO180; however, ZNF304 levels were significantly higher in SKOV3IP1 cells. Silencing ZNF304 inhibits migration and proliferation in OC cells Given the potential role of ZNF304 in cancer metastasis, we next investigated whether silencing this target would affect invasion and migration. We first tested the knockdown efficiency of three siRNA sequences of ZNF304 in HeyA8 cells ( Supplementary Fig. 3 ). Two of the three siRNA sequences tested (ZNF304 siRNA-1 and ZNF304 siRNA-3) showed more than 65% inhibition of ZNF304 in HeyA8 cells. Therefore, these two siRNA sequences were selected for further studies. Next, we performed invasion and migration assays in HeyA8 and SKOV3IP1 cell lines with the selected siRNA sequences, resulting in 40% inhibition of invasion and 45% inhibition of migration in HeyA8 cells ( Fig. 2a,b , respectively) and 27% inhibition of migration in SKOV3IP1 cells ( Fig. 2c ). 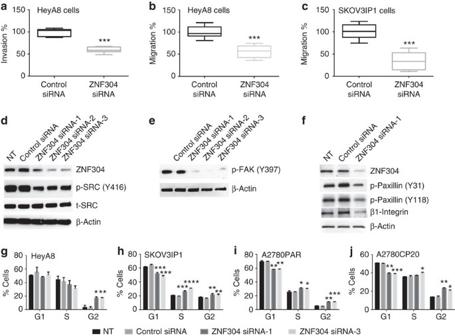Figure 2: Silencing ZNF304 inhibits migration and proliferation. The effect of ZNF304 silencing on invasion % (a), migration % (b) of HeyA8 cells and migration % of SKOV3IP1 cells (c). Migration and invasion percentages in ZNF304 siRNA-treated samples were calculated after normalization with control siRNA-treated samples. Box-and-whisker plots showing median (horizontal line), interquartile range (box) and maximum/minimum range (whiskers). All images shown are representative of three independent experiments and data are presented as mean±sem of n>3 experimental groups. *P≥0.05,**P≥0.01 and ***P≥0.001 (Student’st-test). (d) Western blot analysis of ZNF304, p-Src (Y416) and total src levels 72 h post transfection with all ZNF304 siRNA sequences in HeyA8 cells. (e) Levels of focal adhesion kinase phosphorylation (Y397) after ZNF304 downregulation by all ZNF304 siRNA sequences in HeyA8 cells. (f) Immunoblotting results of β1 integrin and p-paxillin (Y31) and p-paxillin (Y118) after 72 h of ZNF304 siRNA treatment in HeyA8 cells. Cell-cycle arrest analysis of HeyA8 cells (g), SKOV3IP1 cells (h), A2780PAR cells (i) and A2780P20 cells (j) after 72 h transfection with ZNF304 siRNA. Cells were harvested at 72 h and were fixed, stained with propidium iodide and analysed by fluorescence-activated cell sorting. Data are presented as the percentage of cells as mean±s.e.m.ofn≥3 experimental groups. *P≥0.05, **P≥0.01,***P≥0.001 (Student’st-test). Figure 2: Silencing ZNF304 inhibits migration and proliferation. The effect of ZNF304 silencing on invasion % ( a ), migration % ( b ) of HeyA8 cells and migration % of SKOV3IP1 cells ( c ). Migration and invasion percentages in ZNF304 siRNA-treated samples were calculated after normalization with control siRNA-treated samples. Box-and-whisker plots showing median (horizontal line), interquartile range (box) and maximum/minimum range (whiskers). All images shown are representative of three independent experiments and data are presented as mean±sem of n>3 experimental groups. * P ≥0.05,** P ≥0.01 and *** P ≥0.001 (Student’s t -test). ( d ) Western blot analysis of ZNF304, p-Src (Y416) and total src levels 72 h post transfection with all ZNF304 siRNA sequences in HeyA8 cells. ( e ) Levels of focal adhesion kinase phosphorylation (Y397) after ZNF304 downregulation by all ZNF304 siRNA sequences in HeyA8 cells. ( f ) Immunoblotting results of β1 integrin and p-paxillin (Y31) and p-paxillin (Y118) after 72 h of ZNF304 siRNA treatment in HeyA8 cells. Cell-cycle arrest analysis of HeyA8 cells ( g ), SKOV3IP1 cells ( h ), A2780PAR cells ( i ) and A2780P20 cells ( j ) after 72 h transfection with ZNF304 siRNA. Cells were harvested at 72 h and were fixed, stained with propidium iodide and analysed by fluorescence-activated cell sorting. Data are presented as the percentage of cells as mean±s.e.m.of n ≥3 experimental groups. * P ≥0.05, ** P ≥0.01,*** P ≥0.001 (Student’s t -test). Full size image To determine the potential signalling pathways in which ZNF304 is involved, we performed a reverse phase protein array (RPPA) analysis of control siRNA-treated and ZNF304 siRNA-treated HeyA8 cells. Samples were probed with 214 validated antibodies to total proteins and the respective phospho-proteins. Silencing ZNF304 led to reduced expression of caveolin-1, fibronectin, MYH9 (myosin II) and the effectors of the Ras signalling pathway (BRAF, RAF1; Supplementary Fig. 4 ). This last finding guided us to further analyse the link between ZNF304 and integrin signalling ( Supplementary Table 1 ). ZNF304 mRNA expression was highly correlated with β1 integrin expression in HGSOC samples ( r =0.20, P =0.0015; Spearman’s rank-order correlation test, Supplementary Fig. 5 ). To further understand the role of ZNF304, we validated the RPPA data and determined the levels of focal adhesion complex members after ZNF304 siRNA transfection in HeyA8 cells. Silencing ZNF304 decreased phosphorylation of Src and FAK, which are adaptor proteins of focal adhesion and major markers of cell migration ( Fig. 2d,e , respectively). To further analyse pathways related to migration and invasion, we investigated the effects of ZNF304 silencing on paxillin and β1 integrin ( Fig. 2f ). ZNF304 silencing inhibited both paxillin phosphorylation at tyrosine sites 31 and 118 and β1 integrin expression in the cell lines tested. In the RPPA results, forkhead box M1 (FOXM1) and cyclin B1 levels were also decreased in ZNF304-silenced samples, suggesting that ZNF304 might play a role in the cell cycle. To determine the effects of ZNF304 silencing on proliferation, we performed cell-cycle analysis in HeyA8, SKOV3IP1, A2780PAR and A2780CP20 cell lines after 72 h of ZNF304 siRNA transfection ( Fig. 2g–j , respectively). All cell lines treated with ZNF304 siRNA showed significant arrest in the G2 phase, confirming the decreases in cyclin B 1 and FOXM1 levels found in the RPPA analysis. ZNF304 transcriptionally regulates β1 integrin The ZNF304 gene is located at chromosome 19q13.43 ( http://www.genome.ucsc.edu ). The ZNF304 protein consists of a Kruppel-associated box domain and 16 zinc finger proteins (UniProt; Supplementary Fig. 6 ). To explore the mechanism by which ZNF304 silencing downregulates migration, we determined protein and mRNA levels of β1 integrin upon ZNF304 siRNA treatment in HeyA8 and SKOV3IP1 cells. We first performed reverse transcription–PCR (RT–PCR) and real-time RT–PCR to determine the effects of the selected ZNF304 siRNA sequences on ZNF304 mRNA levels; the results showed the downregulation of ZNF304 mRNA in these cells ( Supplementary Fig. 7a,b , respectively). We also determined reduced β1 integrin mRNA levels after ZNF304 silencing using real-time RT–PCR ( Supplementary Fig. 7c,d ). We determined the basal protein levels of β1 integrin and observed that it was expressed in the cell lines tested ( Fig. 3a ). 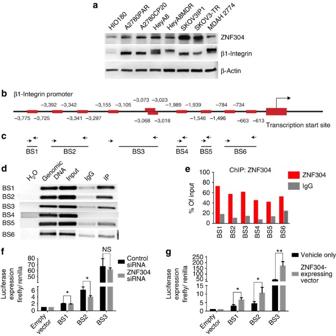Figure 3: ZNF304 associates with ITGB1 promoter and regulates β1 integrin expression. (a) Western blot analysis of basal protein expression levels of ZNF304 and β1 integrin in HIO180 (non-transformed ovarian cell line) and six ovarian cancer cell lines. (b) The ten predicted binding sites of ZNF304 in the ITGB1 promoter on the basis of support vector machine scores using an online tool, which is available athttp://compbio.cs.princeton.edu/zf/. (c) ITGB1 promoter with ten predicted binding sites (in red) and six primer sets were designed for the ten predicted binding sites. (d) Chromatin immunoprecipitation (ChIP) analyses with ZNF304 antibody in HeyA8 cells. Relevant sequences were quantified by PCR with six pre-designed primers subsequent to ChIP assay. (e) Densitometric analysis of ChIP data. Sequence and antibody-specific controls were included. Data are presented as percentage of input. (f) Luciferase activity in control siRNA (black)- or ZNF304 siRNA (grey)-treated HeyA8 cells. Fold induction was calculated after normalization with empty vector. Data are presented as mean±s.e.m. of n≥3 experimental groups. *P≥0.05, **P≥0.01,***P≥0.001 (Student’st-test). Luciferase activity was inhibited after control siRNA treatment or ZNF304 siRNA treatment in BS1-vector-, in BS2-vector- and in BS-3-vector-transfected cells. (g) Luciferase activity increased after transfection of ZNF304-expressing vector into BS1-, BS2- and BS3-vector-transfected HeyA8 cells. Data are presented as mean±s.e.m. ofn≥3 experimental groups. *P≥0.05, **P≥0.01,***P≥0.001 (Student’st-test). NS, not significant. Figure 3: ZNF304 associates with ITGB1 promoter and regulates β1 integrin expression. ( a ) Western blot analysis of basal protein expression levels of ZNF304 and β1 integrin in HIO180 (non-transformed ovarian cell line) and six ovarian cancer cell lines. ( b ) The ten predicted binding sites of ZNF304 in the ITGB1 promoter on the basis of support vector machine scores using an online tool, which is available at http://compbio.cs.princeton.edu/zf/ . ( c ) ITGB1 promoter with ten predicted binding sites (in red) and six primer sets were designed for the ten predicted binding sites. ( d ) Chromatin immunoprecipitation (ChIP) analyses with ZNF304 antibody in HeyA8 cells. Relevant sequences were quantified by PCR with six pre-designed primers subsequent to ChIP assay. ( e ) Densitometric analysis of ChIP data. Sequence and antibody-specific controls were included. Data are presented as percentage of input. ( f ) Luciferase activity in control siRNA (black)- or ZNF304 siRNA (grey)-treated HeyA8 cells. Fold induction was calculated after normalization with empty vector. Data are presented as mean±s.e.m. of n≥3 experimental groups. * P ≥0.05, ** P ≥0.01,*** P ≥0.001 (Student’s t -test). Luciferase activity was inhibited after control siRNA treatment or ZNF304 siRNA treatment in BS1-vector-, in BS2-vector- and in BS-3-vector-transfected cells. ( g ) Luciferase activity increased after transfection of ZNF304-expressing vector into BS1-, BS2- and BS3-vector-transfected HeyA8 cells. Data are presented as mean±s.e.m. of n ≥3 experimental groups. * P ≥0.05, ** P ≥0.01,*** P ≥0.001 (Student’s t -test). NS, not significant. Full size image We next investigated whether ZNF304 transcriptionally regulates β1 integrin. ZNF304-DNA-binding sites were predicted on the basis of support vector machines [11] . We identified ten possible ZNF304-binding sites in the β1 integrin promoter by using support vector machine scores that ranged from 24.25 to 18.9 ( Supplementary Fig. 8 ). The transcription start site was predicted by the ensemble and was compared with the β1 integrin transcript sequence and the binding locations in the β1 integrin promoter region ( Fig. 3b ). Six primer sets containing the segments for the ten binding sites were designed ( Fig. 3c ). DNA segments were amplified, cloned, sequenced and confirmed with a standard nucleotide–nucleotide basic local alignment search tool (National Center for Biotechnology Information). To determine whether ZNF304 binds to the β1 integrin promoter, we performed chromatin immunoprecipitation (ChIP) assays in HeyA8 cells with ZNF304 antibody. Subsequent PCR results confirmed the interaction of β1 integrin promoter and five of the six predicted ZNF304-binding sites (BS1, BS2, BS3, BS5 and BS6; Fig. 3d ). A densitometric analysis of the inputs and immunoprecipitation results for each binding site revealed that BS1, BS2 and BS3 had an affinity of >50% ( Fig. 3e ). Owing to their affinity, BS1, BS2 and BS3 were selected for further studies. To identify the role of ZNF304 in the regulation of β1 integrin gene transcription, we developed three constructs that each contained one of the binding sites and inserted them into pGL3-basic vector. HeyA8 cells were transfected with the constructs, and the activity of each binding site was determined by a dual-luciferase reporter assay in cells with basal ZNF304 expression and in cells in which ZNF304 had been knocked down by siRNA. As shown in Fig. 3f , overall luciferase activity increased in cells transfected with the binding site constructs compared with cells transfected with the empty vector. Cells transfected with BS1-vector had two times more luciferase expression than empty vector cells, whereas BS2-vector-transfected cells had six times more luciferase expression than did the empty vector cells. Cells transfected with BS3-vector showed the highest luciferase activity ( ∼ 70 times more expression than empty vector cells). ZNF304 silencing led to a decrease in luciferase activity in all three binding sites. The most significant was BS2-transfected cells, which had a 40.3% inhibition of luciferase activity ( P= 0.02; Fig. 3f ). We found a 13.8% decrease in luciferase activity for cells transfected with BS1-vector and a 7.8% decrease for cells transfected with BS3-vector, compared with control cells ( P= 0.0173 and P =0.2630, respectively). Co-transfection of ZNF304-expressing vector significantly induced the luciferase activity of BS1-, BS2- and BS3-vector-transfected cells ( Fig. 3g ). These results indicate that ZNF304 is a positive regulator of the active β1 integrin promoter and that ZNF304 increases its transcription by binding to BS2. ZNF304 protects tumour cells from anoikis β1 integrin confers a survival advantage to tumour cells [12] . As a regulator of β1 integrin, ZNF304 can also inhibit anoikis through β1 integrin downregulation. Therefore, we examined the anoikis rates at 24, 48 and 72 h in detached HeyA8 cells in vitro using polyhydroxyethylmethacrylate-coated tissue culture plates that promote anchorage-independent cell growth [13] . The anoikis rates in ZNF304 siRNA-transfected cells were significantly higher than control siRNA-transfected cells at each time point tested (at 24, 48 and 72 h; Supplementary Fig. 9 ). The highest anoikis rate and induction of poly ADP ribose polymerase (PARP) cleavage were observed at 72 h; therefore all subsequent experiments were conducted at this time point. Cells transfected with the ZNF304 siRNAs for 72 h had a significantly higher ( [ZNF304 siRNA-1, P<0.0001]; [ZNF304 siRNA-3, P<0.0005]) rate of anoikis (75–80%), than control untreated or control siRNA-treated cells (60%; Fig. 4a ). Consistent with these results, immunoblotting from these samples showed that silencing ZNF304 also increased PARP cleavage ( Fig. 4b ), which supports our observation of increased anoikis in cells transfected with ZNF304 siRNA. 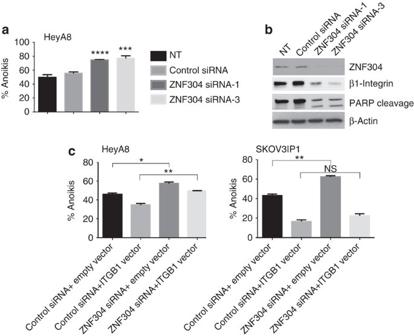Figure 4: ZNF304 mediated inside-out signalling. (a) The anoikis rates of HeyA8 cells at 72 hours post transfection in suspension condition. HeyA8 cells were transfected with indicated siRNAs, and incubated in anoikis plates for 72 h; cells were analysed by flow cytometry following Annexin V-FITC and propidium iodide (PI) staining. Data are presented as mean±s.e.m. ofn≥3 experimental groups. *P≥0.05, **P≥0.01,***P≥0.001, ****P≥0.0001 (Student’st-test). (b) Immunoblotting analysis of HeyA8 cells in suspension conditions at 72 h after treatment with control siRNA or ZNF304 siRNA; followed by protein isolation and immunoblotting. Data are presented as mean±s.e.m. ofn≥3 experimental groups. **P≥0.01,***P≥0.001, ****P≥0.0001 (Student’st-test). Poly ADP ribose polymerase cleavage indicates enhanced anoikis in ZNF304 siRNA-treated and control siRNA-treated samples in suspension conditions. (c) The anoikis rates of HeyA8 and SKOV3IP1 cells in suspension after ZNF304 silencing and β1 integrin overexpression. Cells were analysed by flow cytometry following Annexin V-FITC and PI staining. Data are presented as mean±s.e.m. ofn≥3 experimental groups. *P≥0.05, **P≥0.01,***P≥0.001 (Student’st-test). NS, not significant. Figure 4: ZNF304 mediated inside-out signalling. ( a ) The anoikis rates of HeyA8 cells at 72 hours post transfection in suspension condition. HeyA8 cells were transfected with indicated siRNAs, and incubated in anoikis plates for 72 h; cells were analysed by flow cytometry following Annexin V-FITC and propidium iodide (PI) staining. Data are presented as mean±s.e.m. of n ≥3 experimental groups. * P ≥0.05, ** P ≥0.01,*** P ≥0.001, **** P ≥0.0001 (Student’s t -test). ( b ) Immunoblotting analysis of HeyA8 cells in suspension conditions at 72 h after treatment with control siRNA or ZNF304 siRNA; followed by protein isolation and immunoblotting. Data are presented as mean±s.e.m. of n ≥3 experimental groups. ** P ≥0.01,*** P ≥0.001, **** P ≥0.0001 (Student’s t -test). Poly ADP ribose polymerase cleavage indicates enhanced anoikis in ZNF304 siRNA-treated and control siRNA-treated samples in suspension conditions. ( c ) The anoikis rates of HeyA8 and SKOV3IP1 cells in suspension after ZNF304 silencing and β1 integrin overexpression. Cells were analysed by flow cytometry following Annexin V-FITC and PI staining. Data are presented as mean±s.e.m. of n ≥3 experimental groups. * P ≥0.05, ** P ≥0.01,*** P ≥0.001 (Student’s t -test). NS, not significant. Full size image To determine the link between ZNF304-mediated β1 integrin and anoikis, we also performed a rescue experiment. HeyA8 and SKOV3IP1 cells were transfected with either control siRNA or ZNF304 siRNA. Next, cells were transiently transfected with either empty vector or β1 integrin-expressing vector and transferred to anoikis plates. Both HeyA8 and SKOV3IP1 cells that were transfected with β1 integrin-expressing vector showed increased survival and decreased anoikis rates ( Fig. 4c left and right, respectively). Furthermore, silencing ZNF304 increased the anoikis sensitivity and death rate of HeyA8 cells even in the presence of high β1 integrin expression. In addition, we generated mutations (5 bp deletion on the binding site) on the ZNF304-overexpressing vector that led to insensitivity for ZNF304 siRNA-1 ( Supplementary Fig. 10 ). We performed the rescue experiment using the ZNF304 overexpressing vector and mutant ZNF304-overexpressing vector. Immunoblotting showed that overexpression of mutant ZNF304 (insensitive for ZNF304 siRNA-1) led to a decrease in PARP cleavage, indicating the lack of anoikis in these cells ( Supplementary Fig. 10 ). Sustained in vivo ZNF304 gene silencing On the basis of our in vitro findings, we next investigated whether ZNF304 gene silencing would be effective in treating orthotopic murine models of OC. For the in vivo experiments, we developed and characterized a novel delivery system designed for sustained and prolonged gene silencing. DANPs were prepared by using a chitosan core coated with polylactic acid. These particles had a diameter of 150–200 nm and a zeta potential of −10 mV, which corresponded to a neutral range ( Fig. 5a,b , respectively). Atomic force microscopy images demonstrated the spherical morphology and size distribution of the DANP ( Fig. 5c ). This optimized nanoparticle formulation was used for all subsequent experiments owing to their small size, slight negative charge and high efficiency at incorporating siRNA. We incorporated siRNA in the chitosan core by using chitosan/tripolyphosphate at a 3:1 ratio, which yielded more than 75% loading efficiency, as previously described [14] . We next determined the tissue distribution of the DANP by labelling the particles with rhodamine 6G and administering these red fluorescence-labelled particles as a single dose intravenously to HeyA8 tumour-bearing mice. Twenty-four hours later, the mice were euthanized, and their major organs and the tumours were removed, processed and sectioned. The number of particles in each field was assessed by fluorescence microscopy ( Fig. 5d ). 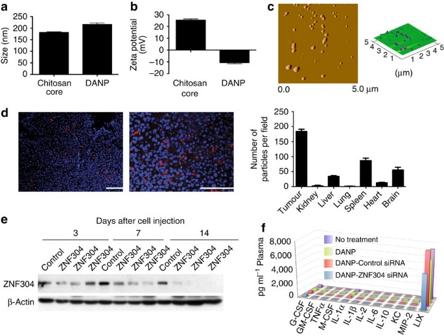Figure 5: Sustainedin vivoZNF304 gene silencing. (a) Size and (b) zeta potential of DANP determined by Zeta Sizer. (c) Atomic force microscopy images of DANP showing the morphology and size distribution of particles. (d) Biodistribution of rhodamine 6G-labelled DANPin vivo. Tumour and the major organs were removed 24 h after a single administration of rhodamine 6G-labelled DANP. The nanoparticles were monitored using fluorescent microscopy and representative images were taken at × 20 (left) and × 40 magnification (centre). Scale bar, 100 μm. Number of nanoparticles was counted at five fields per slide (right). Data are presented as means±standard error of the mean (s.e.m.). (e) Sustainedin vivoZNF304 silencing in HeyA8 orthotopic model of OC. Tumours were removed and analysed by immunoblotting at 3, 7 and 14 days after a single administration of DANP-Control siRNA or DANP-ZNF304 siRNA. (f) Effect of DANP, DANP-Control siRNA and DANP-ZNF304 siRNA on cytokine levels in plasma at 72 h, after a single intravenous administration. Inflammatory cytokine responses were assessed in the serum of C57 black mice. Mice were treated with single i.v. injections of DANP alone (n=6), DANP-Control siRNA (n=6), DANP-ZNF304 siRNA (n=6) and no treatment (n=2), and serum was collected after 72 h using cardiac puncture. A Luminex assay designed to detect 12 pro-inflammatory cytokines was used. Figure 5: Sustained in vivo ZNF304 gene silencing. ( a ) Size and ( b ) zeta potential of DANP determined by Zeta Sizer. ( c ) Atomic force microscopy images of DANP showing the morphology and size distribution of particles. ( d ) Biodistribution of rhodamine 6G-labelled DANP in vivo . Tumour and the major organs were removed 24 h after a single administration of rhodamine 6G-labelled DANP. The nanoparticles were monitored using fluorescent microscopy and representative images were taken at × 20 (left) and × 40 magnification (centre). Scale bar, 100 μm. Number of nanoparticles was counted at five fields per slide (right). Data are presented as means±standard error of the mean (s.e.m.). ( e ) Sustained in vivo ZNF304 silencing in HeyA8 orthotopic model of OC. Tumours were removed and analysed by immunoblotting at 3, 7 and 14 days after a single administration of DANP-Control siRNA or DANP-ZNF304 siRNA. ( f ) Effect of DANP, DANP-Control siRNA and DANP-ZNF304 siRNA on cytokine levels in plasma at 72 h, after a single intravenous administration. Inflammatory cytokine responses were assessed in the serum of C57 black mice. Mice were treated with single i.v. injections of DANP alone ( n =6), DANP-Control siRNA ( n =6), DANP-ZNF304 siRNA ( n =6) and no treatment ( n =2), and serum was collected after 72 h using cardiac puncture. A Luminex assay designed to detect 12 pro-inflammatory cytokines was used. Full size image In our first set of experiments, we determined the duration of in vivo DANP-mediated ZNF304 silencing in an orthotopic HeyA8 mouse model. DANP-ZNF304 siRNA (300 μg kg −1 body weight) was administered as a single intravenous injection 2 weeks after tumour inoculation. Groups of mice were euthanized on day 3, 7 and 14 after injection. Tumours were collected and analysed by immunoblotting to determine ZNF304 protein expression levels. We demonstrated that ZNF304 protein silencing started at day 3 and continued up to 14 days after a single administration of DANP-ZNF304 siRNA ( Fig. 5e ). Next, inflammatory cytokine responses were assessed in the serum of C57 black mice. Mice were treated with single i.v. injections of DANP alone ( n =6), DANP-Control siRNA ( n =6), DANP-ZNF304 siRNA ( n =6) or no treatment ( n =2; Fig. 5f ), and serum was collected after 72 h using cardiac puncture. A Luminex assay designed to detect 12 pro-inflammatory cytokines (LIX, MIP-2, KC, interleukin (IL)-10, IL-6, IL-2, IL-1β, IL-1α, macrophage colony-stimulating factor (CSF), tumour-necrosis factor α, granulocyte–macrophage CSF, granulocyte-CSF) was used. The results obtained did not show any significant increase in these cytokines. Tissue samples were also obtained for post-mortem histopathology studies (brain, spleen, liver and kidney). Haematoxylin and eosin staining of the various tissues were analysed by our Histopathology Core’s veterinary pathologist; no inflammatory changes were observed in the tissues studied ( Supplementary Fig. 12 ). Blood chemistries to assess liver (ALT and Alk Phosp) and kidney function (BUN and S. Creatinine) were also conducted ( Supplementary Fig. 11 ); haematologic profile was conducted (Complete Blood Counts, with differential and platelets: Hgb, Hct including red blood cell parameters are shown in Supplementary Table 2 ). All parameters studied were within normal range. Furthermore, tissue assessment using haematoxylin and eosin did not disclose any toxicity. ZNF304 gene silencing leads to antitumour activity On the basis of these findings, we examined the antitumour activity of weekly or biweekly ZNF304 silencing in two orthotopic OC mouse models, HeyA8 and SKOV3IP1. In the first model, mice were injected with HeyA8 cells to induce tumours and 1 week later they were randomly assigned to six treatment groups (ten mice in each group): DANP alone, DANP-Control siRNA, DANP-ZNF304 siRNA (150 μg kg −1 body weight) administered weekly, DANP-ZNF304 siRNA (300 μg kg −1 body weight) administered biweekly, as paclitaxel is commonly used for OC treatment and combines effectively with many biologically targeted agents, paclitaxel only or a combination of paclitaxel plus DANP-ZNF304 siRNA (300 μg kg −1 body weight, biweekly administration; Fig. 6a ). Significant reductions in tumour weight were observed in the groups treated with DANP-ZNF304 siRNA weekly or biweekly. Mice treated with DANP-ZNF304 siRNA had a significantly lower tumour burden (62% reduction in tumour weight; P <0.01; Fig. 6a , left panel) and had 50% fewer nodules than did mice treated with DANP-Control siRNA ( P <0.05; Fig. 6a , right panel). Moreover, the DANP-ZNF304 siRNA treatment group had significantly fewer nodules than did the control group ( P =0.0001, weekly administration; P =0.0001, biweekly administration; Student’s t -test). 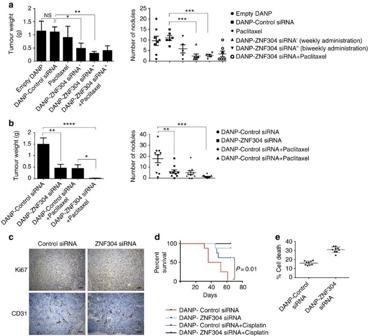Figure 6: Effects ofin vivoZNF304 gene silencing on tumour growth and vasculature. (a) Effect of ZNF304 siRNA-DANP treatment on tumour weight (left panel) and number of nodules (right panel) in HeyA8 orthotopic murine model (Pvalues obtained with Student’st-test; *P<0.05; **P<0.01; ***P<0.001 or ****P<0.0001; compared with control siRNA-treated group; bars and error bars represent mean values and the corresponding s.e.m). (b) Knockdown of ZNF304 by DANP-ZNF304 siRNA and the effect of treatment in SKOV3 tumour weight (left) and number of nodules (right). Data are presented as mean± s.e.m. (n=10 per group). *P<0.05; **P<0.01; ***P<0.001 or ****P<0.0001 (Student’st-test). (c) Immunohistochemical stainings for tumour proliferation (Ki67) and microvessel density (CD31) in SKOV3 orthotopic murine model of OC. Scale bar, 100 μm. Quantification of Ki67-positive and CD31-positive cells in control siRNA and ZNF304 siRNA-treated groups are shown inSupplementary Fig. 14. (d) Kaplan–Meier survival curve illustrating the effects of DANP-ZNF304 siRNA treatment versus control siRNA treatment for thein vivoOVCA-432 survival model. Survival curves indicate that biweekly treatment of DANP-ZNF304 siRNA improves survivalin vivo(n=8 per group,P=0.01 (Control siRNA versus ZNF304 siRNA), Log-rank (Mantel-Cox) test). (e) Viability of epithelial cells in ascites of mice. DANP-siRNA was administered intravenously when ascites was detectable. Ascites was removed 7 days after a single administration and viability of epithelial cells were detected by FITC-Epcam and PI staining followed by flow cytometry (n=3,P<0.0001, Student’st-test). NS, not significant. Figure 6: Effects of in vivo ZNF304 gene silencing on tumour growth and vasculature. ( a ) Effect of ZNF304 siRNA-DANP treatment on tumour weight (left panel) and number of nodules (right panel) in HeyA8 orthotopic murine model ( P values obtained with Student’s t -test; * P <0.05; ** P <0.01; *** P <0.001 or **** P <0.0001; compared with control siRNA-treated group; bars and error bars represent mean values and the corresponding s.e.m). ( b ) Knockdown of ZNF304 by DANP-ZNF304 siRNA and the effect of treatment in SKOV3 tumour weight (left) and number of nodules (right). Data are presented as mean± s.e.m. ( n =10 per group). * P <0.05; ** P <0.01; *** P <0.001 or **** P <0.0001 (Student’s t -test). ( c ) Immunohistochemical stainings for tumour proliferation (Ki67) and microvessel density (CD31) in SKOV3 orthotopic murine model of OC. Scale bar, 100 μm. Quantification of Ki67-positive and CD31-positive cells in control siRNA and ZNF304 siRNA-treated groups are shown in Supplementary Fig. 14 . ( d ) Kaplan–Meier survival curve illustrating the effects of DANP-ZNF304 siRNA treatment versus control siRNA treatment for the in vivo OVCA-432 survival model. Survival curves indicate that biweekly treatment of DANP-ZNF304 siRNA improves survival in vivo ( n =8 per group, P =0.01 (Control siRNA versus ZNF304 siRNA), Log-rank (Mantel-Cox) test). ( e ) Viability of epithelial cells in ascites of mice. DANP-siRNA was administered intravenously when ascites was detectable. Ascites was removed 7 days after a single administration and viability of epithelial cells were detected by FITC-Epcam and PI staining followed by flow cytometry ( n =3, P <0.0001, Student’s t -test). NS, not significant. Full size image In the second orthotopic model (SKOV3IP1), the treatment groups were (i) DANP-Control siRNA, (ii) DANP-ZNF304 siRNA, (iii) DANP-Control siRNA plus paclitaxel and (iv) DANP-ZNF304 siRNA plus paclitaxel ( n =10 per group). DANP-siRNA was administered intravenously every 2 weeks in all treatment groups. Tumours removed from mice treated with DANP-ZNF304 siRNA alone weighed 60% less than those of mice treated with DANP-control siRNA ( Fig. 6b , left panel). Number of nodules was dramatically reduced in mice treated with either DANP-ZNF304 siRNA or DANP-ZNF304 siRNA plus paclitaxel ( Fig. 6b , right panel). The greatest reduction was observed in the group treated with both DANP-ZNF304 siRNA and paclitaxel. None of the groups in either mouse model showed decreased body weight, which indicates that the treatments were not toxic ( Supplementary Fig. 13 ). These data indicate that inhibiting ZNF304 results in antitumour activity in mouse models of OC and that the DANP delivery system is an efficient tool for in vivo gene silencing. Given the in vitro effects of ZNF304 silencing, we performed Ki67 and CD31 staining to examine the biological effects of silencing ZNF304 on tumour cell proliferation and angiogenesis, respectively. Mice treated with DANP-ZNF304 siRNA showed significant reduction in cell proliferation compared with control group ( P <0.0001; Fig. 6c ). Given that ZNF304 transcriptionally regulates β1 integrin, which is required for endothelial cell adhesion, migration and survival [16] , [17] , we also examined the effects of ZNF304 siRNA treatment on angiogenesis. The DANP-ZNF304 siRNA treatment group had significantly reduced microvessel density compared with the control ( P =0.0252, Students’s t- test; Supplementary Fig. 14 ). These data showed that downregulation of ZNF304 was highly associated with decreased cell proliferation and decreased microvessel density. On the basis of efficacy data, we next examined the effects of DANP-ZNF304 siRNA treatment on tumour-bearing mice survival. For these experiments, mice inoculated with OVCA-432 cells that represent HGSOC [18] . Luciferase-labelled OVCA-432 cells (3 × 10 6 ) were injected intraperitoneally to generate tumours in nude mice. The four groups ( n =8 per group) were treated with either: (i) DANP-Control siRNA, (ii) DANP-ZNF304 siRNA, (iii) DANP-Control siRNA+cisplatin and (iv) DANP-ZNF304 siRNA+cisplatin. The treatment started 1 week after the tumour cell inoculation and the mice were monitored daily by three observers. Individual mice were euthanized on the day the core veterinarian recommended, based on moribund status. A Kaplan–Meier curve was generated based on the survival duration of mice ( Fig. 6d ). DANP-ZNF304 siRNA-based treatment significantly improved survival compared with DANP-Control siRNA treatment ( n =8 per group, P =0.01, Log-rank test). Our analysis showed that the median survival for DANP-Control siRNA-treated group was 44 days, whereas it was not reached for the DANP-ZNF304 siRNA. Next, we addressed whether ZNF304 silencing could directly increase the rates of anoikis in vivo . For this question, we use the OC MDAH 2774 cell line as it induces significant ascites in mice [13] . MDAH 2774 cells were implanted into the peritoneal cavity of nude mice, and ascites production was observed 4–6 weeks post inoculation. Next, we analysed the ascites for viable tumour epithelial cells using fluorescein isothiocyanate (FITC)-labelled anti-epithelial cellular adhesion molecule antibody followed by flow cytometry analysis ( Fig. 6e ). The control group showed 16% (mean±s.e.m. ; 16.08±0.7280, n =3) epithelial cell death in ascites, whereas mice treated with intravenous DANP-ZNF304 siRNA had up to 30% (mean±s.e.m. ; 30.77±1.040, n =3) epithelial cell death. These results show that silencing ZNF304 significantly decreased the ability of OC cells to survive in ascites ( P <0.001, Student’s t -test). The key finding from this study is that ZNF304 is a novel transcriptional regulator of β1 integrin. Silencing ZNF304 resulted in antitumour activity and the induction of anoikis in malignant cells both in vitro and in vivo through β1 integrin downregulation. High ZNF304 mRNA expression was associated with worse survival in OC patients. Furthermore, silencing ZNF304 enhances the anoikis rate through inhibiting inside-out integrin signalling and accordingly blocking outside-in signalling ( Fig. 7 ). 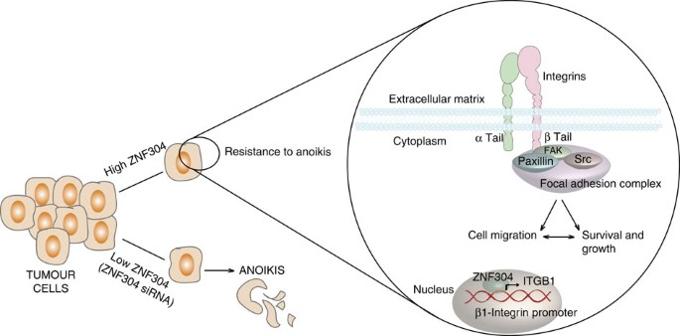Figure 7: A schematic representation of mechanisms by which ZNF304 downregulation enhances anoikis in tumour cells. The model illustrates that silencing ZNF304 leads to anoikis in tumour cells, whereas high-ZNF304-expressing cells gain resistance to anoikis through increased integrin β1 expression and activation of focal adhesion complex members. Figure 7: A schematic representation of mechanisms by which ZNF304 downregulation enhances anoikis in tumour cells. The model illustrates that silencing ZNF304 leads to anoikis in tumour cells, whereas high-ZNF304-expressing cells gain resistance to anoikis through increased integrin β1 expression and activation of focal adhesion complex members. Full size image Integrins are crucial for normal functions of multicellular organisms and critical at each step of cancer: tumorigenesis, progression and metastasis [19] . Integrins are regulated and activated by conformational changes, clustering and trafficking [20] . These transmembrane proteins are an essential link between the extracellular matrix (ECM) and the cytoplasm, and the signalling can be in two directions: outside-in or inside-out through the cytoplasmic β tail [20] . For example, β1 integrin promotes cell survival and regulates focal adhesion, leading to tumour metastasis in many types of cancer including OC [21] , [22] , [23] , [24] . In a recent study, Schiller and colleagues demonstrated that expression of α5β1 integrins is essential to sense the stiffness of fibronectin-based ECM, which is also critical for tumour metastasis [25] , [26] . Furthermore, several β1 integrin-targeting strategies, such as monoclonal antibodies and peptide inhibitors, showed activity in clinical trials for cancer therapy [19] , [27] , [28] . However, targeting ZNF304—the regulator of β1 integrin expression—may offer greater efficacy than targeting only activation of β1 integrin. β1 integrin is a subunit of heterodimeric membrane adhesion receptors, and it can form heterodimers with integrin α subunits. For example, α4β1, α8β1 and αvβ1 are fibronectin-binding integrins; α3β1, α6β1 and α7β1 interact with laminin and nectin; and α1β1, α2β1, α10β1 and α11β1 bind to collagens [29] , [30] . The first study showing the inside-out regulation of β1 integrin unraveled the control by R-Ras of the ligand-binding affinity of β1 integrin and fibronectin [31] . Thus, the regulation of integrin activation and affinity was known as a transcription-independent function of the Ras-linked mitogen-activated protein kinase pathway [32] , [33] . However, the transcriptional regulation of β1 integrin remained unknown. Here, we elucidated that the regulation of β1 integrin expression through ZNF304 is at transcriptional level. Previous studies showed that fibronectin and β1 integrin ligation, followed by activation of cytoplasmic β subunit, promotes the invasive migration of OC cells through the ECM [34] . Myosin II and FAK mediate the phosphorylation of paxillin, reinforcing the cytoskeletal ECM linkage and driving focal adhesion maturation [35] . In addition, β1 integrin-FAK signalling directs the initial proliferation of micrometastatic cancer cells disseminated in the lungs, which indicates the role of integrin-FAK signalling in the metastatic cascade [36] . Thus, ZNF304 may be a regulator of this metastatic process. Correspondingly, we showed that silencing the key regulator ZNF304 decrease nodule formation, tumour growth and prolong survival in orthotopic mouse models of OC. The functional crosstalk between cell adhesion receptors and receptor tyrosine kinases contributes to cancer cell survival [22] . The interaction between ErbB1 and β1 integrin induces tumour cell detachment, migration and metastatic potential. β1 integrin was also shown to regulate epidermal growth factor receptor signalling in lung cancer cells [37] and to mediate epidermal growth factor-induced cell invasion in OC cells [38] . Furthermore, a recent study demonstrated an increased ErbB1-β1 integrin heteroassociation in high-grade astrocytomas and showed that this clinically relevant association can be targeted by molecular therapy [39] . Therefore, silencing ZNF304—the regulator of β1 integrin—may also inhibit epidermal growth factor receptor signalling, inhibiting cancer cell survival and slowing tumour progression. Anoikis is a form of apoptosis in adherent nonmalignant cells caused by a lack of integrin-mediated survival signals from the ECM [40] , [41] . However, malignant cells develop resistance to anoikis, leading to increased metastatic potential [42] , [43] . A seminal mechanistic work on anoikis unraveled its contribution to human cancer metastasis in several different malignancies [44] , [45] , [46] . Integrins are crucial in anoikis mechanism as major mediators of adhesion between cells and ECM proteins [47] , [48] . A recent study showed that activated integrins enhance the metastatic potential of prostate cancer cells by decreasing their sensitivity to anoikis during tumour dissemination and by increasing their interactions with ECM ligands during extravasation [49] . This latter study suggested that in prostate cancer cells, β1 integrin is activated through an inside-out signalling, which also enhances its affinity for ligand binding. The interaction of β1 integrin with ECM ligands further activates β1 integrin through outside-in signalling. RNA interference is a highly effective method for gene silencing owing to its sequence specificity; however, systemic delivery of RNA interference remains a challenge. Our group has previously developed and characterized chitosan nanoparticles for systemic delivery of siRNA [14] , [50] . Although chitosan nanoparticles is an efficient RNA interference delivery system, weekly administration is required as the target downregulation lasts only for 7 days after a single administration. Thus, DANP prolonged silencing is a more tolerable and promotes patient compliance. Integrative computational analysis and patient data selection Clinical and expression data (Level 3 Illumina HiSeqv2) for 260 patients were downloaded from TCGA portal and were used to analyse the relationship between expression of ZNF304 and overall survival as well as between expressions of ZNF304 and ITGB1. The Spearman’s rank-order correlation test was applied to measure the strength of the association between ZNF304 and ITGB1 levels in patient samples in TCGA data set. Cell lines and culture The immortalized non-transformed human ovarian surface epithelial cell line HIO-180 and the human epithelial OC cell lines HeyA8, MDAH 2774, SKOV3IP1, A2780PAR and A2780CP20 were maintained as described previously [51] , [52] , [53] , [54] , [55] . Taxane-resistant HeyA8MDR and SKOV3-TR cells were maintained in Roswell Park Memorial Institute 1640 medium supplemented with 10% fetal bovine serum and 0.1% gentamicin sulfate (Gemini Bio-Products) with or without paclitaxel (300 ng ml −1 for HeyA8-MDR; 150 ng ml −1 for SKOV3-TR). The A2780CP20 cell line was developed by sequential exposure of the A2780 cell line to increasing concentrations of cisplatin. All of the cell lines are routinely screened for Mycoplasma species (Mycoalert Mycoplasma Detection Kit, Lonza). All in vitro and in vivo experiments were conducted when cells were 70–80% confluent. Western blot analysis Western blot analysis was performed as previously reported [56] , [57] . All antibodies used in this study and vendors are listed in Supplementary Table 4 . Uncropped scans of the western blot results are shown in Supplementary Figs 15–18 . SiRNA constructs and delivery SiRNAs were purchased from Qiagen or Sigma-Aldrich. A non-silencing siRNA that did not share sequence homology with any known human mRNA was used as a control for target siRNA. In vitro transient transfection was performed as described previously [56] . The ZNF304 and control siRNA sequences are listed in Supplementary Table 3 . Invasion and migration assays Cell migration and invasion assays have been described previously [58] , [59] . For migration/invasion assays, cells were treated with either control or ZNF304 siRNA for 48 h and incubated on migration wells for 24 h. Migrated cells on the bottom of the wells were collected, fixed, stained and counted by light microscopy. Cells were counted in ten random fields ( × 200 final magnification), and the average number of migrated cells was calculated; the percentage of migration was determined by setting control siRNA-treated samples as 100% migration/invasion. RPPA This study was conducted at the University of Texas MD Anderson Cancer Center RPPA Core Facility [60] . First step was to denature cellular proteins in 1% SDS lysis buffer containing β-mercaptoethanol. This was followed by serial dilutions (two- to fivefold serial dilutions). Next, the lysates were arrayed on the nitrocellulose-coated slides (Grace Bio-Labs). On each slide 5,080 spots were arranged. The spotted samples were arrayed with an Aushon 2,470 arrayer (Aushon BioSystems). Only validated primary antibodies with a correlation Pearson’s Coefficient of greater than 0.7 were used in the RPPA analysis. Signals were amplified using a Dako Cytomation-catalysed system (Dako) and visualized by diaminobenzidine colorimetric reaction. To generate the spot intensity, customized software was used (MicroVigene, VigeneTech Inc.). Dilution curves were fitted with a logistic model (‘Supercurve Fitting’ developed by the Department of Bioinformatics and Computational Biology in MD Anderson Cancer Center, ‘ http://bioinformatics.mdanderson.org/OOMPA ’). Both observed and fitted curves were plotted on the y axis and the log2-concentration of proteins on the x axis. Protein concentrations for each set were normalized by Tukey’s median polish, corrected across samples by linear expression values using the median expression levels of all antibody experiments to calculate a loading correction factor for each sample. Cell-cycle analysis Cells were transfected with either control siRNA or ZNF304 siRNA, trypsinized and collected 72 h post transfection. Samples were washed in PBS solution and were fixed in 75% ethanol overnight. Cells were then centrifuged and reconstituted in PBS with propidium iodide (PI; 50 μg ml −1 ), as previously described [61] . PI fluorescence was assessed by flow cytometry, and the percentage of cells in each cycle was analysed by FlowJo software. Chromatin immunoprecipitation assay HeyA8 cells were cultured in 10% fetal bovine serum to ∼ 75% confluence, and cells were cross-linked with 37% formaldehyde for 20 min and were incubated with glycine (0.125 M) as previously described [62] . Cells were lysed, and chromatin was sonicated according to the protocol provided by the kit (EZ ChIP, Upstate Biotechnology; cat #17-371). Possible binding sites of ZNF304 in the ITGB1 promoter were predicted using an online tool ( http://compbio.cs.princeton.edu/zf/ ). Six primer pair sets were designed using basic local alignment search tool software (National Center for Biotechnology Information). Primers used for amplification of the DNA in quantitative PCR are shown in Supplementary Table 5 . Anti-ZNF304 antibody ( Supplementary Table 4 ) was used for the chromatin immunoprecipitation assays. The Bio-Rad DNA Engine Dyad Thermal Cycler (Bio-Rad) was used with the following cycling conditions: 2 min at 94 °C, followed by 35 cycles of 30 s at 94 °C, 30 s at 58 °C and 1 min at 68 °C, followed by 1 min at 68 °C. Plasmid construction and luciferase reporter assay Fragments containing the predicted binding sites (BS1, BS2 and BS3) were amplified from HeyA8 cell genomic DNA by PCR using primers containing Sac I or Hin dIII restriction enzyme sites. The PCR products were purified, digested and subsequently cloned into the same restriction site of the pGL3 control vector (Promega) downstream of the firefly luciferase reporter gene. Sequences were analysed with a DNA BigDye Terminator sequencing kit, version 3.1 (Life Technologies). HeyA8 cells were plated in 24-well plates (60,000 cells per well) 24 h before transfection with either ZNF304 siRNA or ZNF304-expressing vector (Promega). Twenty-four hours after the first transfection, cells were transfected with the luciferase reporter vectors containing BS1, BS2 or BS3 together with Renilla luciferase construct, which was used as a normalization reference. Transfections were performed with Attractene transfection reagent (Qiagen) according to the manufacturer’s instructions. Cells were lysed 48 h after luciferase vector transfection, and activity was measured using a dual-luciferase reporter assay system (Promega) in the Veritas microplate luminometer (Turner BioSystems). Three independent experiments were performed in technical triplicates. Wild-type vectors for ZNF304 (gene ID: 57343) and ITGB1 (gene ID: 16412) were purchased from Promega (San Luis Obispo, CA). ZNF304 vector was used to generate mutant vector (7-bp deletion) by using the QuikChange Site-Directed Mutagenesis Kit (Agilent Technologies) using the primers in Supplementary Table 5 . In vitro anoikis Cells were transfected with control or ZNF304 siRNA and transferred to six-well tissue culture plates that were coated with polyhydroxyethylmethacrylate, and cells were cultured in these plates for 72 h at 37 °C in a 5% carbon dioxide atmosphere. Cells were washed with PBS and were stained with Annexin V-FITC and PI solution (50 μg ml −1 ) containing RNase A (25 μg ml −1 ). After incubating the pellets for 30 min at 37 °C, we analysed cell viability by flow cytometry. Preparation of DANP DANPs were prepared via ionic gelation of anionic tripolyphosphate and siRNA. Briefly, predetermined tripolyphosphate (0.25%, weight/volume) and siRNA (1 μg μl −1 ) were added to chitosan solution, and the siRNA/chitosan nanoparticles spontaneously formed under constant stirring at room temperature. After incubating the nanoparticles at 4 °C for 40 min, we collected the siRNA/DANP by centrifugation (Heraus Biofuge Fresco) at 16,000 g for 40 min at 4 °C. Chitosan nanoparticles were coated with polylactic acid polymer under probe sonication, and the organic solvent was evaporated. The pellet was washed in sterile water three times to isolate siRNA/DANP, which was stored at 4 °C until used. For the biodistribution study, DANPs were labelled with rhodamine 6G (Sigma-Aldrich). Rhodamine 6G (0.1%, weight/volume) was added to the polymer solution (chloroform) in the simple emulsion. The particles were collected and were washed three times to eliminate the nonencapsulated marker. Orthotopic in vivo models of OC and tissue processing Female athymic nude mice (NCr-nu; 8–12 weeks old) were purchased from the National Cancer Institute-Frederick Cancer Research and Development Center (Frederick, MD) and were maintained as previously described [56] . The MD Anderson Cancer Center Institutional Animal Care and Use Committee approved and supervised all animal studies. Mice were cared for in accordance with guidelines set forth by the American Association for Accreditation of Laboratory Animal Care and the United States Public Health Service Policy on Human Care and Use of Laboratory Animals. To generate tumours, SKOV3IP1 cells (1 × 10 6 ), HeyA8 cells (2.5 × 10 5 ) or (3 × 10 6 ) OVCA-432 cells were injected into the peritoneal cavity, as previously described [63] . For therapy experiments, ten mice (eight mice per group for OVCA-432 in vivo study) were assigned randomly to each group. This sample size was sufficient to provide 80% power for a test at significance level of 0.05. Treatments with control or ZNF304 siRNA incorporated in DANP were intravenously administered either weekly (150 μg kg −1 body weight) or biweekly (300 μg kg −1 body weight). Paclitaxel (100 μg per mouse for the HeyA8 model and 75 μg per mouse for the SKOV3 model) was injected intraperitoneally once weekly. Mice were euthanized 6 weeks after first administration in SKOV3 model and 4 weeks after first administration in HeyA8 model. After euthanasia, we recorded mouse and tumour weight, number of nodules and distribution of tumours. Individuals who performed the necropsies were blinded to the treatment group assignments. Tissue specimens were fixed with either formalin or optimal cutting temperature medium (Miles) or were snap-frozen in liquid nitrogen. For OVCA-432 survival study, the treatment started 1 week after the tumour cell inoculation and the mice were monitored daily by three observers. Individual mice were euthanized on the day the core veterinarian recommended, based on moribund status. For the biodistribution study of DANP, mice were injected peritoneally with HeyA8 cells (2.5 × 10 5 ) for tumour inoculation. When tumours were detectable, rhodamine 6G-labelled particles that contained control siRNA (150 μg kg −1 ) were administered intravenously. After 24 h, mice were euthanized; tumours and the major organs (brain, heart, kidney, spleen, liver and lungs) were removed and fixed in optimal cutting temperature medium and sectioned. The organ and tumour distribution of particles were assessed by fluorescence microscopy. In vivo anoikis Viability of tumour cells from ascites fluid was determined by dual staining with PI and epithelial cell adhesion molecule tagged with FITC. MDAH 2,774 cells (2 × 10 6 ) were injected intraperitoneally into nude mice, and treatments started when mice developed detectable ascites. Mice were divided into two groups ( n =3 per group), receiving a single administration of either DANP-control siRNA or DANP-ZNF304 siRNA (300 μg kg −1 ). After 7 days, ascites fluid was drawn from the peritoneal cavity and rapidly centrifuged at 500 g for 10 min. Pellets were washed with a red blood cell lysis buffer and reconstituted in PBS. Suspended cells were then incubated with excited state absorption-FITC (1:30 dilution) for 30 min at room temperature. After incubation, cells were washed and stained with a PI solution (50 μg ml −1 ). Cells were then incubated for 30 min at 37 °C and analysed on a Gallios flow cytometer (Beckman Coulter). Immunohistochemical analysis Analyses of tumours cell proliferation and microvessel density were conducted by following procedures described previously [14] , [64] , [65] . Two investigators quantified the number of positive cells in a blinded manner. The antibodies used and the vendors are listed in Supplementary Table 4 . Statistical analysis Unless specified otherwise, all data are presented as the mean values±the standard error of the mean from at least three independent experiments. Two-sided t -tests were used to test the relationships between the means of data sets, and P values indicate the probability of the means compared, being equal with * P <0.05, ** P <0.01 and *** P <0.001. Student’s t -tests and analysis of variance were calculated with GraphPad software. Statistical analyses were performed in R (version 3.0.1; http://www.r-project.org/ ), and P values less than 0.05 were considered statistically significant. For the analysis of RPPA results, we used the Benjamini–Hochberg multiple testing correction [66] to estimate the false discovery rate. How to cite this article: Aslan, B. et al. The ZNF304-integrin axis protects against anoikis in cancer. Nat. Commun. 6:7351 doi: 10.1038/ncomms8351 (2015).